Direct imaging of Joule heating dynamics and temperature profiling inside a carbon nanotube interconnect Understanding resistive (or Joule) heating in fundamental nanoelectronic blocks, such as carbon nanotubes, remains a major challenge, particularly in regard to their structural and thermal variations during prolonged periods of electrical stress. Here we show real-time imaging of the associated effects of Joule heating in the channel of carbon nanotube interconnects. First, electrical contacts to nanotubes entirely filled with a sublimable material are made inside a transmission electron microscope. On exposure to a high current density, resistive hotspots are identified on (or near) the contact points. These later migrate and expand along the carbon nanotube, as indicated by the localized sublimation of the encapsulated material. Using the hotspot edges as markers, it is possible to estimate the internal temperature profiles of the nanotube. Simple and direct, our method provides remarkable spatial and temporal insights into the dynamics of resistive hotspots and millisecond-paced thermal variations occurring inside nanoscaled tubular interconnects. Interconnects, that is the connecting unit between two active components, are key elements of any electrical circuit or electronic device [1] . Commonly made of metallic wires, much effort has been dedicated to understand how to best contact them to electrodes and preserve their structural integrity when exposed to the continuous electrical stress typical of device operation [2] . Translating this knowledge into nanoelectronic devices is essential, but serious obstacles exist due to the minimal dimensions involved [3] , [4] , [5] , [6] , [7] . One-dimensional nanostructures, such as carbon nanotubes (CNTs), have emerged as promising building blocks for next-generation electronic devices owing to their potential for size miniaturization, faster responses and superior energy efficiency [8] . Recently, following the report of a thermally actuated CNT nanodevice [4] , there has been much interest on the thermal gradients induced by the exposure of a nanotube to high electrical current densities [5] , [6] . Static temperature profiling along a single, electrically heated CNT has been realized [6] . Logically, the next step towards a comprehensive description of electrical heating in CNTs is the study of the dynamics of heat transfer along and across these materials, as well as its effect on the internal channel. Here we followed the entire operating life cycle of a CNT-electrode circuit with high spatial and temporal resolutions. Using a transmission electron microscope (TEM), we imaged the dynamical events associated with Joule heating inside a CNT from the moment the contacts were established to the final electrical breakdown of the interconnect. Interestingly, we find that, during the first stages of electrical contact, the channel temperature in the nanotubes is not necessarily maximal at the contact location and that the subsequent evolution of the resistive hotspot can result in not just longitudinal thermal gradients but also in radial ones. Joule heating dynamics To evaluate the heat-transfer process, a sample of CNTs entirely filled with a lower vapour pressure material was used, Zn 0.92 Ga 0.08 S@CNT (where @ stands for encapsulated in). More details on the sample can be found in the Supplementary Figures S1-S3 and Supplementary Table S1 . The electrical circuit was mounted within a TEM sample holder ( Supplementary Fig. S4 ) and designed in two different contact modes, that is, the CNT was connected either by its ends or its sidewalls ( Fig. 1 ). Once assembled, an increasing bias was slowly applied to promote Joule heating and controllably remove the chalcogenide filling. 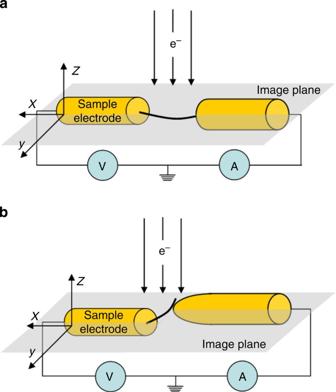Figure 1: Schematics of the two electrical contact modes used to follow the Joule heating dynamics. Using the nanomanipulator integrated in the TEM holder, the freestanding Zn0.92Ga0.08S@CNT located at the sample electrode was gently pressed against the counter electrode. Both electrodes were bare-metal Au (or W) wires. (a) An end-contact configuration where the CNT is connected at both ends. (b) A side-contact configuration where the two electrodes are connected to the CNT wall. In both modes the CNT is under electron beam (e−) illumination and its ends are on the same z-height (image plane). Figure 1: Schematics of the two electrical contact modes used to follow the Joule heating dynamics. Using the nanomanipulator integrated in the TEM holder, the freestanding Zn 0.92 Ga 0.08 S@CNT located at the sample electrode was gently pressed against the counter electrode. Both electrodes were bare-metal Au (or W) wires. ( a ) An end-contact configuration where the CNT is connected at both ends. ( b ) A side-contact configuration where the two electrodes are connected to the CNT wall. In both modes the CNT is under electron beam (e − ) illumination and its ends are on the same z-height (image plane). 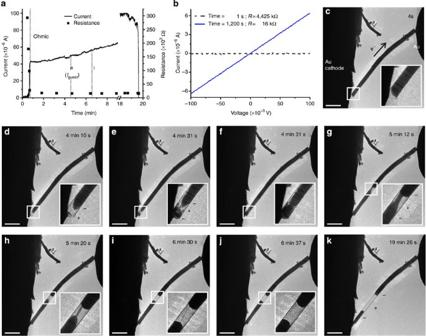Figure 2: Correlated electrical and structural behaviour of a sulphide-filled CNT interconnect. The electrically induced core removal process is tightly linked to the resistive hotspot dynamics and takes place in three well-defined stages: hotspot generation, migration and expansion. (a) Current passing through the nanotube and corresponding electrical resistance during the removal process shown in (c–k). The steep increase at ~40 s occurs when an Ohmic contact is established. The dotted vertical lines mark the corresponding position of panels (e) and (i). Elimination of the applied bias led to the abrupt fall in current at ~20 min. (b) Current–voltage relations taken at the initial and final stages of the removal process. A change from an almost insulating to an Ohmic system is visible and concurs with the event seen at ~40 s in (a). (c) Initial configuration of an isolated Zn0.92Ga0.08S@CNT connected to two Au electrodes. The insets in (c–j) are magnified views of the boxed regions. Plus and minus signs refer to temperatures above and below the sublimation point of the core sulphide, respectively. (d) The first stage of the removal process occurs selectively at one of the CNT ends and refers to the hotspot generation. Localized depletion of the core is evident from (c) to (d). (e–g) During the second stage, and past theIguest=48 μA, the hotspot migrates to a position that is about one-third of the length between the two contact points. This process occurs in a matter of seconds and involves reversible solid–vapour phase transitions happening inside the CNT. (h–k) In the third stage, two core segments are progressively consumed by the expansion of the hotspot. Each segment front acts as a marker for the sulphide sublimation temperature (928 K). All scale bars, 0.5 μm. Full size image Figure 2 illustrates the simultaneous electrical and structural variations taking place inside a filled nanotube interconnect (end-contact configuration) while its core is being removed by passing an electrical current (see also Supplementary Movies 1 and 2 ). The carbon shell has a diameter of about 130 nm with a wall thickness of 5 nm and length of 3.1 μm. This corresponds to a total internal volume of 3.51×10 7 nm 3 and a confined sulphide mass of 143 fg (assuming the gravimetric density of hcp -ZnS, 4.09 g cm −3 ). Figure 2: Correlated electrical and structural behaviour of a sulphide-filled CNT interconnect. The electrically induced core removal process is tightly linked to the resistive hotspot dynamics and takes place in three well-defined stages: hotspot generation, migration and expansion. ( a ) Current passing through the nanotube and corresponding electrical resistance during the removal process shown in ( c – k ). The steep increase at ~40 s occurs when an Ohmic contact is established. The dotted vertical lines mark the corresponding position of panels ( e ) and ( i ). Elimination of the applied bias led to the abrupt fall in current at ~20 min. ( b ) Current–voltage relations taken at the initial and final stages of the removal process. A change from an almost insulating to an Ohmic system is visible and concurs with the event seen at ~40 s in ( a ). ( c ) Initial configuration of an isolated Zn 0.92 Ga 0.08 S@CNT connected to two Au electrodes. The insets in ( c – j ) are magnified views of the boxed regions. Plus and minus signs refer to temperatures above and below the sublimation point of the core sulphide, respectively. ( d ) The first stage of the removal process occurs selectively at one of the CNT ends and refers to the hotspot generation. Localized depletion of the core is evident from ( c ) to ( d ). ( e – g ) During the second stage, and past the I guest =48 μA, the hotspot migrates to a position that is about one-third of the length between the two contact points. This process occurs in a matter of seconds and involves reversible solid–vapour phase transitions happening inside the CNT. ( h – k ) In the third stage, two core segments are progressively consumed by the expansion of the hotspot. Each segment front acts as a marker for the sulphide sublimation temperature (928 K). All scale bars, 0.5 μm. Full size image When a small forward bias was applied along the CNT, an initial current flow of a few nA was detected ( Fig. 2a ). At this point, the current–voltage ( I – V ) curve was characteristic of an almost insulating system ( Fig. 2b ). As seen in Figure 2c , the nanotube is entirely filled and constitutes the sole electrical conduction path between the two Au electrodes. Both ends are clearly visible with their contacts to the metal surfaces being exclusively made at the carbon shell. This shields the semiconductor core from direct contact to the electrodes. With the continued increase of applied bias an Ohmic contact is obtained, confirmed by a strong surge in the electrical current readings (~40 s in Fig. 2a ). The shift in electrical response was further corroborated by the current–voltage ( I – V ) curve taken after the core removal process ( Fig. 2b ). Further bias increments originated structural modifications to the encapsulated material. At first, the sulphide is selectively removed from the areas nearer to the CNT end contacted to the cathode ( Fig. 2d ) by means of a solid-to-vapour phase transition (which explains the presence of the sharp, edged core tip). When the current flow reached 48 μA (4 min 31 s) the response of the interconnect changed. A considerable amount of material was transferred, in less than 1 s, from the core wire to the CNT end where it solidified and accumulated. Immediately, a void was noticeable at the core–shell interface, which moved steadily towards the anode ( Fig. 2e,f , best seen in Supplementary Movie 1 ). This fast mass transfer and void displacement, the second stage of the core removal process, are both ascribed to the migration of a resistive hotspot from the end to a more centred region of the CNT. The onset of these events defines the 'guest threshold current' ( I guest ) of the system. The void commonly stabilizes at one-third to mid-length of the CNTs ( Fig. 2g ). The localization of the hotspot is followed by its expansion, the third stage of the process. Widening of the gap between the two core segments required a current flow of 51 μA. However, this amperage had to be continuously increased to keep the process active (at an average rate of 4 μA min −1 ). To preserve the carbon shell ( Supplementary Fig. S5 ), the current was limited to a maximum of 100 μA during the forward bias run. In the end ( Fig. 2k ), 7.98×10 6 nm 3 of sulphide was sublimed from the CNT (23% of the initial volume, equivalent to 33 fg). A simple calculation of the dissipated power ( P ) and thermodynamics pertaining to the Zn 0.92 Ga 0.08 S@CNT interconnect in Figure 2 explains the solid-to-vapour phase transition. Assuming the molecular weight of ZnS ( M =97.5 gmol −1 ), 143 fg of confined sulphide are equivalent to 1.47×10 −15 mol. Given that the lattice energy of ZnS [9] is −3,561×10 3 J mol −1 , then approximately 5.2×10 −9 J would be sufficient to sublime and ionize the whole extension of the filling. Therefore, as the energy (heat) distribution is longitudinally anisotropic during the electrical heating, it is logical that the first CNT inner-wall region to reach the ~10 −9 J figure is where the phase transition will start. Knowing that, for an Ohmic resistor, the relation P = V × I is applicable and that I guest =48 μA for a voltage of 0.77 V, the maximum dissipated power at the onset of the hotspot migration was 37 μW (the power curve for the whole process is given in Supplementary Fig. S6 ). Thus, at the I guest , an estimated 3.7×10 −5 J was dispersed by the system at each second, a figure four orders of magnitude higher than that necessary to fully sublime the chalcogenide. In these circumstances, it is safe to assume that the retracting segment fronts observed in Figure 2 define the zones within the nanotube channel where the temperature is equivalent to the sublimation point ( T sub ) of the ternary alloy. Ex situ heating experiments, performed in the absence of electrical currents and under inert atmosphere (Ar, 200 Pa), showed that 923 K< T sub (Zn 0.92 Ga 0.08 S) <948 K ( Supplementary Fig. S7 ). Additional 80 kV in situ TEM experiments (vacuum, ~10 −5 Pa) concur, pointing to 928(±10)K. For this reason, we claim that the onset of the structural changes in the internal channel provides a reliable temperature marker ( T =928 K). The forward bias run was promptly followed by an analogous experiment in the reverse regime. Overall, changing the bias direction ( Supplementary Fig. S8 ) led to an adjustment of the hotspot position and its further expansion, but did not result in the generalized reversal of mass transfer observed for metal-filled CNTs and characteristic of electromigration processes [10] , [11] . Further experiments working solely within the reverse or forward regimes (that is, non-cycled) showed similar responses to that seen in Figure 2 . To verify whether the behaviour of the hotspot would be independent of the type of contact, an alternative arrangement and chemistry of the electrodes were explored. 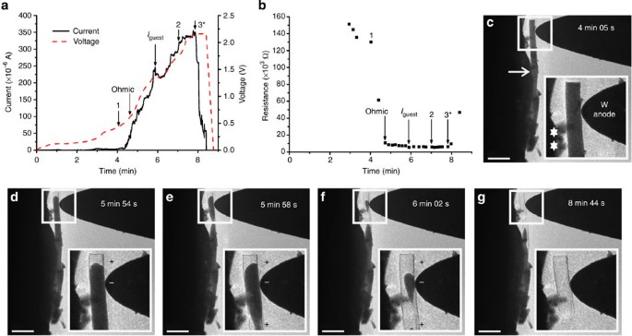Figure 3: Correlated structural and electrical behaviour for a side-contact full life cycle. (a) Chronological evolution of the current (and voltage) flowing through the nanotube. Point 3 is starred as it indicates the onset of visible shell degradation. (b) Time-resolved resistance variations of the system. A minimum is attained immediately after theIguest(246 μA), whereas thinning of the CNT leads to increased values of resistance. (c–g) Collection of video frames representative of the core removal progression (forward bias, Au–W electrodes). The process was performed until the total collapse of the carbon shell. The arrow in (c) indicates the contact point of the suspended CNT section to the supporting Au wire. The particles marked with stars in the inset of (c) are in a different image plane from the CNT and never come in contact with it. The plus and minus signs mark the zones in the carbon shell above and below the sublimation temperature of the sulphide core, respectively. All scale bars, 0.5 μm. The full life cycle (from contact to breakdown) of a Zn 0.92 Ga 0.08 S@CNT under a two-terminal side-contact configuration and corresponding current–voltage, electrical resistance and structural evolution is shown in Figure 3 . Again, the hotspot progressed in three distinguishable stages: formation, migration and expansion ( Fig. 3c–f and Supplementary Movie 3 ). Interestingly, its formation did not take place at the contact point, but at the open tip of the nanotube. This indicates that the hotspot onset within the CNT channel is not necessarily correlated with the contact point. Instead, it appears that the dominant factor is the lattice discontinuity and the presence of the highly irregular structure of the open tips. The localization of the hotspot away from the contact point also confirms that the heat transfer is more efficient longitudinally than transversally. Figure 3: Correlated structural and electrical behaviour for a side-contact full life cycle. ( a ) Chronological evolution of the current (and voltage) flowing through the nanotube. Point 3 is starred as it indicates the onset of visible shell degradation. ( b ) Time-resolved resistance variations of the system. A minimum is attained immediately after the I guest (246 μA), whereas thinning of the CNT leads to increased values of resistance. ( c – g ) Collection of video frames representative of the core removal progression (forward bias, Au–W electrodes). The process was performed until the total collapse of the carbon shell. The arrow in ( c ) indicates the contact point of the suspended CNT section to the supporting Au wire. The particles marked with stars in the inset of ( c ) are in a different image plane from the CNT and never come in contact with it. The plus and minus signs mark the zones in the carbon shell above and below the sublimation temperature of the sulphide core, respectively. All scale bars, 0.5 μm. Full size image Temperature profiling The texture of turbostratic nanotubes is characterized by many intershell interactions and pronounced presence of defects, hence explaining their finite energy dissipation capacity and diffusive conductor characteristics [7] . Furthermore, despite the low efficiency of transversal heat transfer, multi-walled CNTs can function as boilers for encapsulated materials when subjected to high current densities [12] . In the present case, the extension and rate of the phase transitions are closely related to the thermal gradients present along and across the filled CNT. If the removal rate is fast then the CNT will not be able to promptly dissipate the heat and the hotspot will expand uniformly along the nanotube (blunt segments fronts). Oppositely, slow rates (usually <2 μA min −1 ) allow for better heat dissipation, which makes the hotspot front radially anisotropic. This is reflected in the fine structural elements produced inside the CNT. Following analogous studies for externally decorated CNTs [3] , [4] , we used the sulphide fronts as markers to estimate the temperature profiles and thermal gradients both along and across the CNTs. Indeed, and to our best knowledge, experimental probing of the radial heat distribution inside CNTs has never been reported. 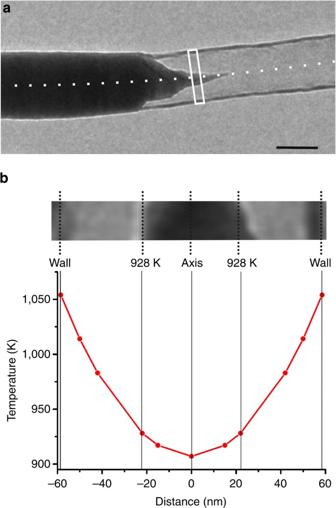Figure 4: Estimate of the radial temperature profile in an electrically heated CNT channel. (a) Section of a partially empty Zn0.92Ga0.08S@CNT showing a sharp conical needle. The dotted line marks the nanotube main axis. The box encloses the area where the temperature profile was estimated from. Scale bar, 100 nm. (b) Plot of the temperature variation across the nanotube's channel. The image at the top corresponds to the box in (a). The sublimation temperature of the sulphide is coincident with the surface layers of the conical needle. Figure 4a shows a section of a 2.82 μm long CNT with a confined thin needle. Under electrical heating, and assuming a parabola-shaped thermal profile for the nanotube cross-section, the maximum temperature in the channel will be located at the inner CNT wall (the cross-shell heat distribution is irrelevant here) and the minimum at the CNT axis (dotted line). Focusing on the boxed area in Figure 4a , the temperature at the needle surface layers should be around 928 K (we predict a maximum error of 5% due to the electron beam effect). Using a longitudinal thermal gradient of 0.7 K nm −1 , it is possible to extract a self-consistent expression that describes the heat distribution across the interior of the carbon shell (details in Supplementary Methods ): Figure 4: Estimate of the radial temperature profile in an electrically heated CNT channel. ( a ) Section of a partially empty Zn 0.92 Ga 0.08 S@CNT showing a sharp conical needle. The dotted line marks the nanotube main axis. The box encloses the area where the temperature profile was estimated from. Scale bar, 100 nm. ( b ) Plot of the temperature variation across the nanotube's channel. The image at the top corresponds to the box in ( a ). The sublimation temperature of the sulphide is coincident with the surface layers of the conical needle. Full size image In this ( x , T) curve, x stands for the shortest distance of a point across the channel to the CNT axis. The second term is a constant that corresponds to the temperature at the axial point. From here, we estimate that the inner wall was at 1,054 K and a radial thermal gradient of 2.5 K nm −1 existed. The corresponding plot is given in Figure 4b . In addition to cross-sections, the outlined methodology can be applied longitudinally. Overall, approximate temperatures and thermal gradients inside a CNT can be simply and rapidly inferred, at any given moment of the electrical-heating process. Taken together, our observations shed light not just on where Joule heating occurs but also on how it evolves inside a nanotubular interconnect subjected to prolonged electrical stress. As the hotspot behaviour for the Zn 0.92 Ga 0.08 S@CNT system is mostly independent of the current flow direction and configuration of the contacts, a common mechanism for the Joule heating dynamics inside a turbostratic CNT can be proposed. 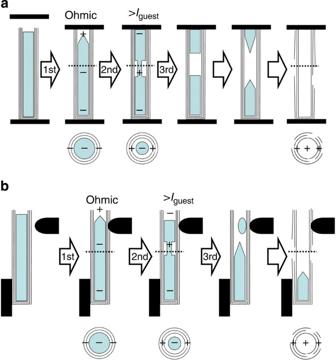Figure 5: Mechanism of Joule heating dynamics inside a filled CNT interconnect. (a) End-contact configuration. (b) Side-contact mode. The plus and minus signs correspond to the areas above and below the core sublimation point, respectively. The dotted lines mark the points where the cross-section views were considered (shown below the CNT models). On the 1st stage, an Ohmic contact is established and a hotspot is generated at the open CNT end. This leads to the localized core sublimation. When theIguestis reached (2nd), the hotspot migrates to mid-length of the tube. Here, the shell is at high temperature due to resistive heating. The formation of thin core bridges signals the presence of radial thermal gradients. On the 3rd stage, the hotspot expands inducing a longitudinal thermal gradient, which is identified by the retraction of the core segments. Further current injection eventually results in electrical breakdown of the conductive shell. Illustrated in Figure 5 , the first step (1st) is the activation of an Ohmic contact between the carbon shell and the Au (W) metal. At this point, a residual contact resistance is expected, as the contact is not yet fully annealed. With increased current density, and consequent Joule heating, a resistive hotspot originates at the open end of the CNT. Scattering of heat/charge carriers is stronger at the edge due to the high density of defects and discontinuity of the carbon lattice [13] . The open tip remains the highest temperature zone of the channel until the I guest is reached (2nd). Then, the temperature at the outer layers of the turbostratic carbon shell is sufficiently high to thermally weld it to the Au surface [14] at the contact point (re-deposition of the sublimed chalcogenide may aid in this process and contribute to minimize the electrical contact resistance). Immediately after this contact optimization, the end is cooled down due to the heat-sinking action of the metallic electrode. Thereafter, the hotspot is displaced to approximately one-third to mid-length of the two contact points. As the current density is further increased so is the dissipated power and the temperature at the hotspot, leading to its propagation as it pushes the chalcogenide segments fronts towards the contact points (3rd). Under slow removal rates, segment bridges and core needles also develop due to the presence of radial thermal gradients. Figure 5: Mechanism of Joule heating dynamics inside a filled CNT interconnect. ( a ) End-contact configuration. ( b ) Side-contact mode. The plus and minus signs correspond to the areas above and below the core sublimation point, respectively. The dotted lines mark the points where the cross-section views were considered (shown below the CNT models). On the 1st stage, an Ohmic contact is established and a hotspot is generated at the open CNT end. This leads to the localized core sublimation. When the I guest is reached (2nd), the hotspot migrates to mid-length of the tube. Here, the shell is at high temperature due to resistive heating. The formation of thin core bridges signals the presence of radial thermal gradients. On the 3rd stage, the hotspot expands inducing a longitudinal thermal gradient, which is identified by the retraction of the core segments. Further current injection eventually results in electrical breakdown of the conductive shell. Full size image In conclusion, using a two-terminal electrical contacts procedure in an electron microscope, direct imaging of dynamical phenomena associated with Joule heating (such as the generation of hotspots and evolving heat distribution) can be realized for the interior of a tubular interconnect. Simple and intuitive, this life cycle method takes advantage of the differentiated thermodynamics of the core–shell interconnect components and thus it may be extended to evaluate the electrical heating behaviour (and eventually electromigration processes) of other tubular structures hosting lower vapour pressure materials. It may also be used as a test-bed for the study of phase transitions occurring in nanoscaled confined spaces. Sample The filled CNTs, herein designated as Zn 0.92 Ga 0.08 S@CNT, were produced as previously reported [15] and used as-made. The shell is composed of several layers of turbostratic-type (pyrolytic) carbon, which provides an electrical conducting path and elasticity to the structure, while its core is an optically active II–VI semiconductor (structural and chemical characterization details in Supplementary Figs S2 and S3 , respectively). Transmission electron microscope The in situ microscopy studies were performed in a JEOL 3100FEF TEM operated at 300 kV. This instrument has a point resolution of 1.7 Å and is equipped with an energy dispersive X-ray detector. Images were taken using a 2k × 2k charge-coupled device camera and the Digital Micrograph suite. Videos were recorded using a video-screen grabber when Digital Micrograph was being operated in the View mode. Transmission electron microscope sample holder Electrical probing and nanomanipulation experiments were carried out with a Nanofactory Instruments single-tilt scanning tunnelling microscopy–TEM holder. At the beginning of each TEM session, the computer controlling the two-probe set-up was synchronized with the image acquisition workstation. Mechanically cut Au wires and chemically etched W wires, 0.25 mm in diameter, were used as electrodes (in Au–Au or Au–W pairs). The etching procedure has been explained elsewhere [16] , [17] . An extended discussion of the factors guiding the response of Zn 0.92 Ga 0.08 S@CNTs to electrical heating is given in Supplementary Methods . How to cite this article: Costa, P.M.F.J. et al . Direct imaging of Joule heating dynamics and temperature profiling inside a carbon nanotube interconnect. Nat. Commun. 2:421 doi: 10.1038/natcomms1429 (2011).